A chemo-centric view of human health and disease Efforts to compile the phenotypic effects of drugs and environmental chemicals offer the opportunity to adopt a chemo-centric view of human health that does not require detailed mechanistic information. Here we consider thousands of chemicals and analyse the relationship of their structures with adverse and therapeutic responses. Our study includes molecules related to the aetiology of 934 health-threatening conditions and used to treat 835 diseases. We first identify chemical moieties that could be independently associated with each phenotypic effect. Using these fragments, we build accurate predictors for approximately 400 clinical phenotypes, finding many privileged and liable structures. Finally, we connect two diseases if they relate to similar chemical structures. The resulting networks of human conditions are able to predict disease comorbidities, as well as identifying potential drug side effects and opportunities for drug repositioning, and show a remarkable coincidence with clinical observations. Humans, in their daily lives, are exposed to a great variety of chemicals, including drugs and environmental hazards. Therapeutic and adverse effects of these chemicals result from a complex interplay with the human body. It is now recognized that, in most cases, a reductionist viewpoint of such interplay is far from reality. Cumulative evidence shows that even the most thoughtfully specific drugs elicit promiscuous interaction profiles [1] and, accordingly, many adverse chemical events lack a compelling molecular explanation [2] . The emerging opinion is that systems biology strategies—that integrate several layers of detail and complexity— will be necessary to zoom out from a reductionist to a more holistic picture of pharmacology and toxicology [3] . As human biology continues to reveal itself more and more intricate, it is suggestive to realize that much information about the behaviour of a chemical inside our bodies is encoded within a small molecule, with few bonds and atoms. Decoding correlations between the structure of a compound and its activity in biological systems has been a prolific research area, and the major goal of earliest pharmacologists [4] . Unfortunately, such a compound-centred view of phenotypes is blind to molecular mechanisms, lacking theoretical support and, therefore, requiring a considerable amount of bioactivity data. In particular, for humans, experiments to obtain this information cannot be conceived, and the bulk of chemical activity assays is placed several translational steps backward (that is, at the level of single receptor binding), with the consequent reduction of the system complexity. Recent advances in text-mining techniques and subsequent curation efforts are committed to compiling direct human response data from the knowledge accumulated through the years [5] , [6] . Here we benefit from this enterprise to revisit the classical structure–activity relationship notion, this time for a vast and diverse list of human diseases. Concretely, we first delve into chemical structures to identify fragments that are associated with adverse or therapeutic responses. Then, we propose disease models based on these fragments, and assess their predictive efficiency. Finally, we use such models to relate diseases, providing a chemical map of human phenotypes. Several resources exist that contain information on the interaction of small molecules with our health. Most notably, the Comparative Toxicogenomics Database (CTD) [5] is mainly focused on environmental chemicals, and reports curated relationships with a comprehensive list of diseases. Moreover, it classifies disease annotations as ‘Marker/Mechanism’ (M) or ‘Therapeutic’ (T). M refers to a chemical that correlates with the disease (that is, a marker) or may act in its aetiology (that is, a toxin), whereas T indicates that the chemical has a known or a potential therapeutic role in the condition (that is, a drug). By analogy, hereafter we refer to adverse and therapeutic disease outcomes simply as M and T diseases, respectively. Research worldwide is conducted at different levels of detail and, accordingly, CTD curators index publications with a hierarchical organization [7] . For instance, although some reports simply congregate ‘Skin diseases’, others are centred on ‘Dermatomyositis’, and even some are focused on a subtype of this condition called ‘Amyopathic dermatomyositis’. Broad disease terms are obviously associated with more molecules (direct annotations plus those regarding child terms); however, they can involve diverse or more intricate mechanisms. As a consequence, extracting molecular rules for imprecise phenotypes may be as challenging as for very specific cases, where data are scarce. We have explored the disease hierarchy with the intuition that, in between general and specific disease concepts, there will be enough information to learn structure–activity relationships. 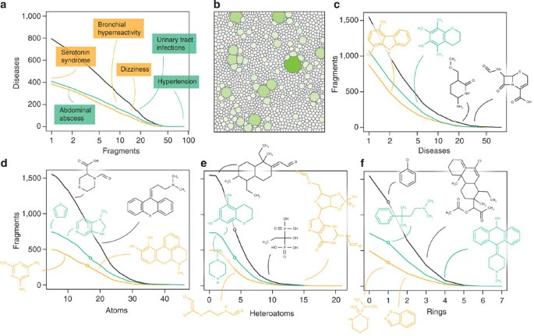Figure 1: Over-represented fragments. Fragments per disease (a) and diseases per fragment (c), considering only the HC set. Inb, a Voronoi diagram where each fragment is a shape with area and colour proportional to the number of molecules that contain it (best match similarity >0.8). To illustrate chemical diversity, we display the cumulative distribution of the total number of atoms (d), the number of heteroatoms (e) and the number of rings (f). Distributions are decorated with illustrative fragment structures. M and T fragment–-disease relationships are shown in orange and green colours, respectively. In total, 934 M and 835 T diseases could be analysed after considering 8,881 molecules ( Table 1 ). These diseases span the medical hierarchy end points, and thus are representative of the variety of known human conditions. Table 1 Disease and fragment statistics. Full size table Chemical fragment mining As a first step in the chemo-centric disease analysis, we sought to list chemical moieties that could be independently associated with the phenotype. Support for this idea is provided by examples of chemical scaffolds showing a strong correlation with bioactivity profiles [8] , [9] . Given, for example, an M set of molecules (that is, biomarkers and toxins of a particular disease), we performed an exhaustive molecular fragmentation and, among the resulting fragments (in this work, the terms ‘fragment’, ‘moiety’, ‘chemotype’ and ‘scaffold’ are used interchangeably), we kept those that were over-represented with respect to compounds unrelated to the disease. We considered non-redundant sets of molecules to minimize annotation biases, and designed the statistical analysis so that the final selection of fragments was simplified in terms of substructural dependencies, without detrimenting posterior predictive models (see Methods). Exactly the same procedure was applied to therapeutic annotations, examining T molecules instead. The median molecule broke into five fragments, ranging from a single piece up to 200. A total of 98,077 moieties were considered. After the significance analysis, both for M and T sets, we obtained around 200 over-represented fragments per disease, and for each fragment, we found four associated diseases. Owing to initial permissive statistical requirements, this constituted a low confidence (LC) set of ~5 × 10 4 fragment—disease associations that was ideal for later achieving predictive power. When we controlled for the false discovery rate below 1% and applied additional constraints (see Methods), we obtained a subset of 7,411 high confidence (HC) fragment—disease pairs ( Supplementary Data 1 ). These fragments are well represented in the known bioactive chemical space ( Supplementary Fig. 1 ), and include both expected and novel moieties, emerging from diverse sets of molecules ( Supplementary Fig. 2 ). Within HC pairs, a fragment was related to a median of 2 M or T diseases, and a disease was linked to six fragments ( Fig. 1a ). At least one HC fragment could be found for 41% and 50% of M and T diseases, respectively ( Table 1 ), providing a chemo-centric molecular description of phenotypes that is interpretable for the medicinal chemist, a property that has been recently vindicated in chemoinformatics [10] . Figure 1: Over-represented fragments. Fragments per disease ( a ) and diseases per fragment ( c ), considering only the HC set. In b , a Voronoi diagram where each fragment is a shape with area and colour proportional to the number of molecules that contain it (best match similarity >0.8). To illustrate chemical diversity, we display the cumulative distribution of the total number of atoms ( d ), the number of heteroatoms ( e ) and the number of rings ( f ). Distributions are decorated with illustrative fragment structures. M and T fragment–-disease relationships are shown in orange and green colours, respectively. Full size image Over-represented fragments in the chemical space Identified fragments exhibit a varied chemical repertoire ( Fig. 1b ). HC moieties have a median size of 17 atoms, including 1 ring and 4 heteroatoms. Interestingly, 32% of the fragments follow the ‘Rule of Three’ (Ro3; molecular weight (MW)<300, number of hydrogen bond donors ≤3, number of hydrogen acceptors ≤3 and logP ≤3). Backward studies found that fragments that accomplish these rules are good starting points to meet the Lipinski condition [11] , or ‘Rule of Five’, that concerns bioavailability of oral drugs (that is, MW<500, hydrogen bond donors ≤5, hydrogen acceptors ≤5 and logP ≤5). Activity-related fragments offer a simple way to compose customized chemical spaces. In Supplementary Data 1 and 2 , they are given together with associated diseases, enabling the design of tailored chemical libraries. In general, although our collection covers a broad and representative spectrum of chemical features, it also reflects the diversity of CTD and most chemogenomics repositories [12] ( Fig. 1a , middle), which contain only a small number of well-represented scaffolds, and a large proportion of singular moieties. The balance between variety of fragments and coverage will depend on the needs. Similar to the case of kinase-focused libraries [13] , we might want to achieve a thorough coverage of a narrow pharmacological space to address, for example, ‘Anterograde Amnesia’, where only two HC fragments represent 55% of the beneficial molecules. Sparse libraries would be preferable in cases like ‘Chronic Obstructive Pulmonary Disease’, where as many as 34 HC fragments can be extracted from the corresponding 27 medicines, spanning 74% of the active space and requiring a higher diversity. Accounting for this diversity is crucial in order to move away from chemical clichés [14] . The structural variety of known drugs [15] and, in general, of registered compounds is very low—the more frequently a scaffold has been used, the more likely it will be used again [16] . However, we have seen that our reported fragments not always emerge from well-studied moieties, yielding valuable novel chemotypes ( Supplementary Fig. 2 ). Recently, it has been suggested that a large part of fragment space is indeed synthetically accessible, which also calls for a more exploratory chemistry [17] . If orphan regions of chemical space are to be populated, we propose that our findings could aid the charting of its biologically relevant, primordial regions. Existence of liable and privileged structures When analysing over-represented structures, the immediate question is whether fragments exist that are mostly associated with adverse events, whereas others are usually present in therapeutic molecules ( Fig. 2a ). The former would correspond to problematic structures that should be avoided in, for instance, medicinal chemistry endeavours [18] . On the contrary, the latter are desired, privileged chemotypes of potential profit in the design of libraries for forward pharmacology practices like cell-based phenotypic screening [19] . 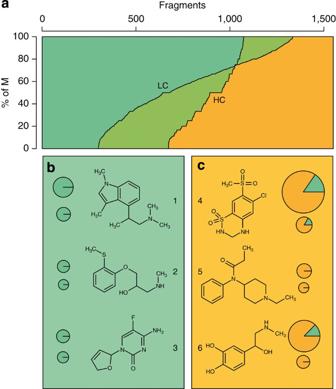Figure 2: Privileged and liable structures. (a) Balance between privileged and liable structures, both for the HC and LC sets. % of M indicates the proportion of M associations for each fragment over its disease associations. (b) Three scaffolds that, while being mostly liable, are included in drug molecules. (c) Fragments that are privileged and remain unsuccessful or unexplored as therapeutics. Next to each structure, top and bottom pie charts represent the number of diseases for which the fragment is LC- and HC-associated, respectively. Area of pie charts is proportional to the number of diseases. To select these examples, experimental and approved drug structures were extracted from Drugbank (July 2013)21. Figure 2: Privileged and liable structures. ( a ) Balance between privileged and liable structures, both for the HC and LC sets. % of M indicates the proportion of M associations for each fragment over its disease associations. ( b ) Three scaffolds that, while being mostly liable, are included in drug molecules. ( c ) Fragments that are privileged and remain unsuccessful or unexplored as therapeutics. Next to each structure, top and bottom pie charts represent the number of diseases for which the fragment is LC- and HC-associated, respectively. Area of pie charts is proportional to the number of diseases. To select these examples, experimental and approved drug structures were extracted from Drugbank (July 2013) [21] . Full size image As expected, it was slightly easier to detect privileged than liable structures (384 versus 367 liable HC fragments, respectively, over a total of 45,607 T and 72,804 M chemical—disease pairs considered ( Table 1 )). The medicinally relevant space is influenced by size constraints and ease of synthesis [20] , and pharmaceutical research is often incremental. Liable fragments, which also occur in drugs and environmental chemicals, may have been abandoned or remained unperceived, and thus are less well represented (Wilcoxon’s test (Wt) P -value <2.2 × 10 −16 ; Supplementary Fig. 3 ). As a consequence, the LC liable fragment occurs in a higher proportion of M compound—disease pairs than the LC privileged fragment in T pairs (Wt P -value 8.0 × 10 −10 ), implying that it might be important across a range of phenotypes, although we can only capture the association with weak statistical signal. On the other hand, as expected, the trend is inverted for HC fragments (Wt P -value 1.4 × 10 −6 ), as only a thorough exploration of chemical space allows for extraction of strong structure–activity relationships. Of particular interests are those privileged fragments that have not been successfully used in drug development yet. Out of the 367 fragments that could be considered as privileged (>80% T both in HC and LC sets), 40% were not present in any approved or experimental drug reported in the DrugBank [21] (note that CTD scope goes beyond drug molecules: 45% of the compounds with T annotations were not found in DrugBank above a similarity cutoff of 0.8). In Fig. 2b , for example, fragment 1 constitutes a fraction of the ergoline tetracycle. Mesulergine is a psychoactive compound of the ergoline class with a halted development because of adverse histological abnormalities in rats [22] . We speculate that 1 , that is present in six other molecules in CTD, could be kept and used to derive safer compounds outside the ergoline family. Fragment 2 is a propanolamine that we found useful to treat ‘Cardiac Arrythmias’ and could be further evolved into Alprenolol alternatives, a close analogue in the market. Finally, 3 is the scaffold of Dexelvucitabine, a failed anti-HIV and anti-HBV agent that, while singular in structure, displays features similar to other desirable chemotypes, and is found over-represented in as many as eight therapeutic indications—safer derivatives of Dexelvucitabine could be of potential interest. Another group of interesting moieties, at least in retrospective, corresponds to those that are frequently included in drug molecules despite being mostly associated with adverse events. We recognize that, in general, drugs (usually prescribed for few indications) will indeed elicit many adverse reactions. However, in CTD the M/T annotation rate is quite balanced (less than 2:1), making >80% M a meaningful definition of a liable fragment. In the right panel of Fig. 2b , structure 4 accounts for the prototypical hydrochlorothiazide, a class that includes methylclothiazide and cyclothiazide. Despite its popularity, we found a large number of adverse events associated to this class, ranging from ‘Hypokalemia’ to ‘Arthritis’. As done elsewhere [23] , 4 could undergo a scaffold-hopping exercise to find better analogues. Fragment 5 , present inside 13 medicines like Sufentanil, constituted a liable HC fragment for five conditions, including ‘Sinus Arrythmia’ and ‘Muscle Hypertonia’. Similarly, 6 is part of several bronchodilator agents and resembles the ancestor Norepinephrine drug. We found eight HC associations of 6 with inconvenient events such as ‘Tachycardia’ and ‘Hypertension’, suggesting that further generations of Norepinephrine successors are likely to remain unsafe. Predictive models Although valuable, identifying the presence of a characteristic fragment in a molecule is usually not enough to accurately infer an association with a disease [24] , [25] . Very often, a combination or mutual exclusion of several moieties will determine the outcome. In general, predictive power and interpretability of structure-activity models are two different objectives that are difficult to achieve simultaneously. On this matter, a good tradeoff is offered by LC fragments, which are more frequent among disease-related molecules, and thus are promising variables for starting machine learning [24] . Given its reduced cost, fragment-based learning can be applied at virtually every step of the drug discovery pipeline, and offers a means to join chemoinformatics with expert opinion [26] . Its performance will largely depend on the specificity of the underlying biology, and the proper, delimited representation of the active chemical space. As a result, although detecting over-represented fragments gets easier for highly annotated, broad disease terms, predictive capability does not follow the same trend ( Supplementary Fig. 4 ). We built a fragment-based chemical classifier for each of the 934 M and 835 T diseases ( Fig. 3 ) using Random Forests (RFs). RFs allow detecting interactions between fragments, for example, when the combination of two fragments has a therapeutic effect but each individual fragment does not. Table 1 provides a general view of the results. It shows, for instance, that point prediction performance metrics sensible to data imbalance (namely, the positive predictive value and the F 1 -score) take values close to zero. This is an expected observation given the pronounced imbalance of positive/unknown sampling (a median of 30:4,250). Also, note that sensitivity could be increased at the expense of the high specificity, and that the decision cutoff could slide at will so that, for example, G -mean is optimized (see Methods). The area under the receiver operating characteristic (ROC) curve (AUC) measures the compromise between sensitivity and specificity at all possible cutoffs, and it is widely used to assess the performance of predictive models. Overall, 184 M and 216 T disease models exhibited a cross-validated AUC above 0.7. The successful models did not display a distinct chemistry ( Supplementary Fig. 5 ), and covered 13% and 7% of the full medical hierarchy end points, respectively. Together, both results evidence our scarce knowledge of the relevant chemical space, and the difficulty to assess a priori if a region of it has been sufficiently exploited. 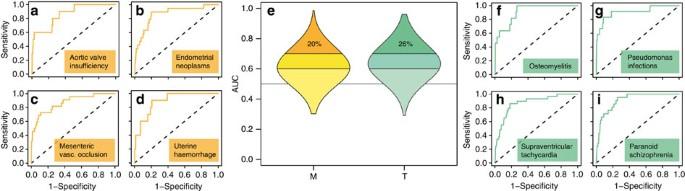Figure 3: Predictive models. AUC distribution of M and T models (e). Area of violin plots is proportional to the number of diseases. Example ROC plots for M and T chemical–disease relationships are shown ina–dandf–i, respectively. Figure 3: Predictive models. AUC distribution of M and T models ( e ). Area of violin plots is proportional to the number of diseases. Example ROC plots for M and T chemical–disease relationships are shown in a – d and f – i , respectively. Full size image Therapeutic effects are better predicted than adverse events When analysing accurate, plausible classifiers ( AUC >0.7), the first observation is that therapeutic outcomes are better modelled than adverse events, that is, there is a larger proportion of T cases with AUC>0.7 (Fisher’s test (Ft) P -value 0.001, and Wt P -value 3 × 10 −8 for whole distributions; Fig. 3 ). Again, this arises from the fact that the therapeutic space is composed of incremental discoveries ( Supplementary Fig. 3 ), and emphasizes the difficulty of the predictive toxicology task. ROC curves on the right of Fig. 3 correspond to satisfactory models of T diseases. ‘Osteomyelitis’, which refers to bone infections, is treated with antibiotics of well-used families (quinolones, cephalosporins, penicillins and so on). Thus, it is easy to infer whether a molecule will be suitable for addressing such condition. A similar chemistry has been learnt for ‘Pseudomonas Infections’, for instance. Analogous conclusions can be drawn for ‘Paranoid Schizophrenia’, where, for example, benzodiazepines and phenothiazines are annotated, and for ‘Supraventricular Tachycardia’, a cardiovascular complication of which the aforementioned propanolamines are prominent examples. Other chemicals, rather than treating, may trigger cardiovascular events. In fact, these are commonly alerted drug side effects. Pergolide, for instance, was withdrawn from the market because of heart issues—we predicted its association with ‘Aortic Valve Insufficiencies’ (this annotation was not available from CTD). A plausible model was also obtained for ‘Mesenteric Valve Insufficiencies’ (left ROC curves in Fig. 3 ). In general, for heart events, even when the underlying biology remains intricate [27] , there is a chemical signal that can aid prevention. In Fig. 3 , we also display the cross-validation of the ‘Uterine Haemorrhage’ model, and, regarding the same organ, that of ‘Endometrial Neoplasms’. Not all types of diseases are equally predictable Following the last example above, we find support for the intuition that travelling the disease hierarchy from specific to broad terms can help to find informative chemical sets. Accordingly, although ‘Neoplasms’ are poorly understood as a whole (AUC=0.66), we obtained a number of accurate models for certain organs and types ( Fig. 4 ). In particular, we could solve many M cancer cases, whereas few successful T models existed. This illustrates that we know more of the chemistry of carcinogens and cancer markers than of the chemistry that is needed to cure it. A similar conclusion could be drawn for ‘Male’ and ‘Female Urogenital Disorders’. On the contrary, we could provide several plausible classifiers for the treatment of ‘Mental Disorders’, meaning that the chemical space that addresses such conditions has been well exploited. Similarly, we have deep knowledge on treating ‘Bacterial Infections and Mycoses’, whereas, as expected, there is little chemistry that may facilitate them (the only example we found was ‘Candidiasis’, where most relevant structures corresponded to steroidal frameworks like glucocorticoids [28] ). The rest of disease classes shared, in general, a balance between M and T plausible models. Remarkably, some disease classes were poorly modelled. We attempted, for instance, 41 M ‘Eye Diseases’, of which as few as 3 yielded a satisfactory classifier. Similarly, we only obtained a good predictor for 4 of the 28 T ‘Endocrine System Disorders’ ( Supplementary Fig. 6 ). 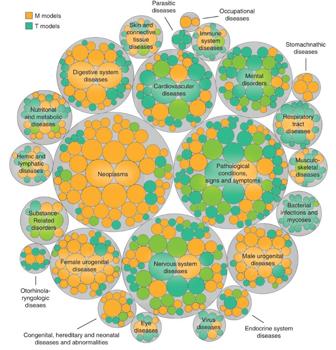Figure 4: Disease categories of successful models. M and T plausible disease models classified in high-level disease categories. Each circle represents an M or T disease model belonging to the corresponding category. Area of circles is proportional to the number of associated molecules in our data set. Figure 4: Disease categories of successful models. M and T plausible disease models classified in high-level disease categories. Each circle represents an M or T disease model belonging to the corresponding category. Area of circles is proportional to the number of associated molecules in our data set. Full size image Indeed, for a majority of diseases we lack an accurate model. We believe, however, that there is room for improving chemical classifiers based on literature mining. One important hindrance in training these classifiers is the absence of truly negative data (chemical—disease pairs that have been verified not to interact, as opposed to not having been observed so far). The so-called ‘positive-unlabelled learning’ tackles this issue and is now being implemented in biomedicine [29] . However, in our hands, such methodologies [30] , [31] did not improve predictive power, most likely due to the sparseness and reduced size of the set of unknowns ( Supplementary Fig. 7 ), an issue that, most likely, will be solved as disease—chemical annotations continue to increase [32] . Also, including physicochemical properties of compounds could be of enormous interest, particularly in the case of adverse events, where mechanisms of action may not be target-driven. Accordingly, the identification of toxicophores is usually thought of in metabolic and reactivity terms [18] , as toxic effects can result from polar or nonpolar processes, uncoupling of oxidative phosphorylation, thiol-alkylation and so on. In this regard, reactivity prediction methods should be appropriate [33] , particularly for nonspecific complications like tissue necrosis, carcinogenicity or immune-mediated toxicities. Recently, a combination of structure and reactivity analysis was applied to select groups that shared structure and electronic state [34] , and it was recommended that compounds undergo a structural clustering before the reactivity assessment, suggesting that our results could be readily complemented with reactivity profiles. Disease networks based on underlying chemistry In this study, we have analysed each disease separately. However, results should be integrated to provide a general view. For this purpose, network representations are a prominent systems biology tool because they integrate relationships between different entities, facilitating contextualization and providing a general view [35] , [36] . In particular, disease networks help to assimilate the diversity of human conditions. In a seminal work, Goh et al. [37] proposed that two diseases could be related if they share a genetic origin. The resulting disease network was able to unveil biological modules and therefore offered a means to link the molecular and the organism levels. Instead of connecting two diseases when the same genes participate in their aetiology, we link them if they relate to a similar chemistry, that is, when the molecules associated with the one are comparable to those associated with the other. The resulting chemo-centric map of human conditions is of singular interest for drug development, as it is focused on intervention, that is, on disease relationships that are directly based on effector compounds. The disease comorbidity network When we relate M disease models, the corresponding network is a comorbidity map, where two conditions are connected if the toxins and markers of the one are similar to those of the other, implying that the two diseases could occur simultaneously. In practice, we screened all M molecule sets annotated to the 934 diseases against the 184 successful M models, and we related two diseases if the AUC of the cross-classification was higher than 0.7. This yielded a network of 12,610 edges ( Table 2 and Supplementary Data 3 ). Interestingly, such a chemo-centric comorbidity map captured disease co-occurrences detected in the history of more than 30 million patients [38] : a medical semantics mapping found that a large number of our disease associations have indeed been observed in the clinics (9,788 matches, the corresponding contingency table yielded a Ft P -value of 4.5 × 10 −28 ), providing an excellent independent validation of our findings (see Methods). For instance, we predicted that molecules associated with ‘Aortic Valve Insufficiency’ are likely related to ‘Neuroleptic Malignant Syndrome’ (AUC=0.88). In turn, the ‘Aortic Valve Insufficiency’ model up-ranked ‘Elimination Disorders’ molecules (AUC=0.82; Fig. 5 ). In patients, not necessarily due to exposure to chemicals, these relationships have been observed with relative risks (RRs) of 56.7 and 29.5, respectively [38] . Overall, together with, for example, studies of metabolic pathways [39] , our results show that a chemical viewpoint is useful to account for the underlying molecular connection of human conditions. Table 2 Network statistics. 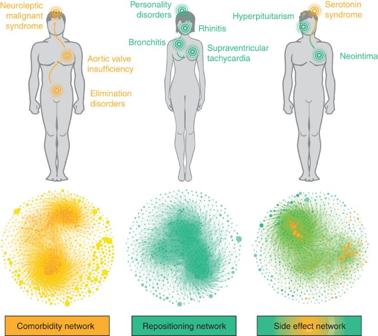Figure 5: Disease networks. Disease comorbidity, drug repositioning and drug side effect networks. Examples discussed in the text are depicted with directed links on top of each network. To select these examples, we looked for strong correlations (see Methods) occurring between diseases in different categories. None of the cases share annotated chemicals, highlighting the value of our fragment-based models. Networks are displayed with a gravity layout, being node size proportional to the number of related chemicals. Network statistics can be found inTable 2. Full size table Figure 5: Disease networks. Disease comorbidity, drug repositioning and drug side effect networks. Examples discussed in the text are depicted with directed links on top of each network. To select these examples, we looked for strong correlations (see Methods) occurring between diseases in different categories. None of the cases share annotated chemicals, highlighting the value of our fragment-based models. Networks are displayed with a gravity layout, being node size proportional to the number of related chemicals. Network statistics can be found in Table 2 . Full size image The drug repositioning network Analogously, we may relate diseases based on T records and obtain a network that links two conditions when medicines for the first could also serve in the second. This so-called ‘drug repositioning network’ is appealing given the time and financial burdens of the drug discovery process. Currently, a number of computational approaches are taken in this direction [40] , and even the simplest methods [41] are proposing remarkable opportunities. After screening the 835 T compound-disease pairs against the 216 good T models, we obtained a network of 14,590 edges ( Table 2 and Supplementary Data 4 ). Some diseases like ‘Hypertension’ had a high in-degree (in this case, 235), meaning that they could be the repurposing opportunity of many indications, reflecting the clinical complexity of this physiological phenomenon associated with cardiovascular, endocrine and nervous system components. On the other hand, ‘Urethral Diseases’ displayed an out-degree of 137, that is, its 11 medicines could have several other uses. When compared with a network drawn from approved indications of drugs [42] , we observed a significant overlap (10,731 common edges, Ft P -value 3.4 × 10 −13 ), reinforcing the validity of our results. This network based on approved drugs represents the polypharmacy of medicines, and links two diseases if they are treated by a significant number of common drugs (see Methods). Even after a conservative semantic mapping, 3,859 of our repositioning opportunities were not found in such network, implying that they remain largely unexplored. Among these, we propose the use of ‘Rhinitis’ therapeuticals like ketotifen for the treatment of ‘Personality Disorders’ (AUC=0.81), and the repurposing of antibronchitic drugs to treat ‘Supraventricular Tachycardia’ (AUC=0.81; Fig. 5 ). The drug side effect network Finally, linking T and M diseases yields a map that relates treatments to potential adverse events. As shown in Table 2 , we screened the 835 T chemical–disease pairs to predict undesired side effects among the 184 M satisfactory models. The resulting network contained as many as 9,921 relationships ( Table 2 and Supplementary Data 5 ). In this network, large peripheral nodes are particularly interesting: ‘Seizures’, for instance, has a well-defined therapeutic chemistry (AUC=0.71) related to as many as 255 molecules, and is not linked to any of the adverse events, suggesting that these treatments are rather safe. When we compared our predictions with side effects extracted from drug package labels [43] , we also observed a significant coincidence (8,686 common associations, Ft P -value=6.9 × 10 −21 ), while still providing 1,235 novel predictions. One of them is the possible appearance of ‘Serotonin Syndrome’ after exposure to ‘Hyperpituitarism’ (for example, carmoxirole) and ‘Neointima’ agents like nebivolol (AUC of 0.78 and 0.81, respectively; Fig. 5 ). Nebivolol, in fact, is metabolized by CYP450 2D6, resembling serotonin reuptake inhibitors—concomitant treatment with such inhibitors may lead to overdose [44] . Overall, these novel associations contribute to the completion of putative drug side effect profiles. In the last years, such profiles have shown useful to elucidate molecular events from phenotypic observations [45] , in turn proving that a lot can still be learnt from the always imperfect drug molecules [46] . Future perspectives The current perception is that systems biology will aid the learning of drug action by rationalizing the influence that small molecules exert on our health [47] . In most cases, drug action is mediated through receptors, being of critical importance their identification. In a previous work [48] , we reported protein targets shared among drugs with a common effect. Our approach was agnostic in the sense that it considered a vast chemical–protein interactome, and was therefore suitable to initiate a systems view. Although we recognize the relevance of target and off-target identification, we found this knowledge insufficient to anticipate side effects, in good agreement with the translational gap in drug discovery [49] . To complement this lack of knowledge, we also mined characteristic chemical moieties inside the drugs with the aim to surrogate phenomena that molecular biology is not yet able to consider, as done by others [50] . We learnt that chemical structures treasure a remarkable predictive power, although they are difficult to inspect given the small number of known drugs and their sparse distribution across the chemical space. Now, our results highlight that collecting and grouping molecules with enough insistency aids the modelling of phenotypic implications with no need to acknowledge all the underlying biological events. Several studies have proven the value of this chemo-centric view of biology. Most notably, such a view allowed for the prediction of ligand binding to protein targets with unresolved structures [51] . Databases like ChEMBL [52] and BindingDB [53] , among others, have been essential to decipher relationships between chemical features and affinity, and a ligand-centred description of the binding event is now feasible [4] . In these databases, hundreds of thousands of distinct compounds are recorded. The ambition to relate chemical structures directly to human-body responses is, undoubtedly, a more challenging task, given the complicated intrinsic biology and the lack of compound records. We have shown that, even when only a few thousand molecules are available, it is already possible to identify scaffolds that correlate and predict phenotypic outcomes. We recognize, however, that scaffold identification is only a starting point, and it may not be sufficient in many cases—ultimately, it will be the modulation of biological networks what determines phenotype, and slight differences in chemical structure may translate into dramatic changes of activity. Moreover, some of the identified scaffolds are the result of follow-on studies and biased reporting systems, narrowing the applicability domain of our method to diseases with varied and abundant annotation of chemicals. Despite these limitations, we anticipate that the number of well-modelled phenotypes could increase considerably in the upcoming years. Concretely, we estimate that the amount of accurate classifiers could be doubled if we would double the annotation of certain diseases ( Supplementary Fig. 8 ). Approximately, increasing by 25% the number of chemical–disease records could result in this doubling of satisfactory models. To guide disease annotators, in Supplementary Data 2, we detail which diseases fall on a learning plateau, be it because they are sufficiently apprehended or largely under-annotated, and which cases will benefit most from curation efforts [54] . Likewise, improving disease annotation will enable the modelling of more specific phenotypes: terms in this study are slightly broader than those commonly used in drug discovery, and these are, in turn, notably unspecific relative to the existing medical vocabulary ( Supplementary Fig. 9 ). To grow the body of chemical records, improvements in text chemical entity identification [55] and new knowledge discovery concepts [56] will be fundamental. Opposite to, for example, genomics, large-scale experimentation in chemistry has been conducted primarily by pharmaceutical industry and, traditionally, proprietary data have not been available to the community. Therefore, scientific literature is still a major support to publish chemical data. We expect that, with the advent of text-mining technologies, resources like CTD will continue to expand in size and scope. Moreover, current chemical–disease records are being gathered together with disease-related genes, which manifests that knowledge is being assembled at a fast pace towards a holistic view of biology. Only now, network-based tools to handle such complexity are flourishing [57] , and urgently demand more chemistry awareness [58] . In this context, our study brings chemical cognizance to the systems level, fulfilling a need of translational sciences, and widening the applicability of network-based strategies. Exhaustive fragmentation Compound structures were obtained by querying the Chemical Identifier Resolver (http://cactus.nci.nih.gov) with CTD names. In addition, we fetched the fraction of chemicals contributed by CTD to PubChem (http://pubchem.ncbi.nlm.nih.gov). Organometallic compounds were excluded, inorganic salts were removed from mixtures and stereochemical information was not considered. In order to include only ‘small molecules’, where fragments would have a similar structural impact, substances with a MW above 800 were also discarded. 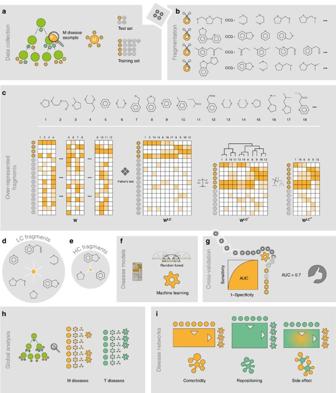Figure 6: Scheme of the method. Analysis protocol exemplified for an M disease of interest. (a) Annotated molecules are collected and split in training and test sets. (b) M training molecules are fragmented using CCQ rules. (c)Wis built from the resulting fragments (columns) and the training set (rows; stratified tenfold cross-validation).Wundergoes a significance filtering, a data balancing step, a column clustering and a pruning, resulting inWLC’. (d) Columns ofWLC’constitute the LC set of fragments; (e) further filtering considering substructural relationships and co-occurrence in molecules yields the HC set. (f) UsingWLC’, a random forest classifier is learnt, and (g) tested against the test set. If the model performs with AUC>0.7, it is considered of good quality. (h) Steps 1–7 are conducted for all M and T chemical–disease relationships. (i) Using plausible models, chemo-centric disease networks are constructed. Figure 6 schemes the processing that these molecules underwent. Figure 6: Scheme of the method. Analysis protocol exemplified for an M disease of interest. ( a ) Annotated molecules are collected and split in training and test sets. ( b ) M training molecules are fragmented using CCQ rules. ( c ) W is built from the resulting fragments (columns) and the training set (rows; stratified tenfold cross-validation). W undergoes a significance filtering, a data balancing step, a column clustering and a pruning, resulting in W LC’ . ( d ) Columns of W LC’ constitute the LC set of fragments; ( e ) further filtering considering substructural relationships and co-occurrence in molecules yields the HC set. ( f ) Using W LC’ , a random forest classifier is learnt, and ( g ) tested against the test set. If the model performs with AUC>0.7, it is considered of good quality. ( h ) Steps 1–7 are conducted for all M and T chemical–disease relationships. ( i ) Using plausible models, chemo-centric disease networks are constructed. Full size image We exhaustively fragmented each chemical structure through recursive bond breaks down to a minimum size of five atoms. We followed JChem’s (http:// www.chemaxon.org ) CCQ fragmentation approach, based on cutting carbon–carbon bonds (CC) if at least one of the carbons is bound to a heteroatom (Q). Thus, CCQ rules do not modify functional groups, ensuring that the resulting fragments conserve the chemical features of the original molecule. Aliphatic rings and aromatic systems were not cleaved either. The 5% of molecules that broke into more than 200 fragments were dismissed. Disease annotation of chemicals We fetched chemical–disease associations from CTD (January 2013) [5] . This knowledgebase includes a controlled vocabulary [7] that is based on the ‘Diseases’ branch of the National Library of Medicine’s Medical Subject Headers (MeSH). MeSH hierarchy grows from broader to more specific disease terms, and molecules are annotated throughout. General concepts include annotations from the more specific ones. To assign M and T molecules to each disease, we fetched curated (‘Direct evidence’) annotations from CTD. Ambiguous annotations (M and T, simultaneously) were removed. Molecules labelled in CTD as ‘inferred’ (through gene—disease triangulation [59] ) were also discarded as they were confounding the obtainment of disease classifiers ( Supplementary Fig. 10 ). The set of ‘unknown’ molecules corresponded to all of those entries that shared no relationship (neither curated nor inferred) with none of the terms in the corresponding branch of the disease vocabulary. Only diseases annotated with at least ten molecules entered further analysis. In total, we kept 934 M and 835 T chemical–disease relationships. To obtain non-redundant sets of chemicals for each disease, we clustered a full pair-wise chemical similarity matrix. Chemical similarity was measured with the widely used topological fingerprints based on hashed molecular sub-graphs, as implemented in the RDKit (http:// www.rdkit.org ). The resulting matrix underwent an unsupervised clustering with the Butina algorithm [60] , which is fast, consistent, parameter free and performs well with hashed fingerprints. Clusters were flattened at a Tanimoto cutoff of 0.8, that is, at a distance of 0.2 to the central molecule. Whenever a disease was associated with several chemicals in a cluster, the molecule with the highest accumulated similarity to the rest was kept as representative for the group. Analogously, we obtained non-redundant sets of disease-unrelated chemicals (unknowns). Fragment mining For each M or T compound–disease pair, we outlined a matrix W listing small molecules in the rows and fragments in the columns. To fill in W , we screened each molecule i against all of the fragments. In a molecule–fragment comparison, we aimed at checking if the molecule contained at least one fragment that was similar to that of interest. This comparison was performed as follows. First, we broke compound i into fragments. Each of the fragments in the resulting set was compared with fragment j . The score of the molecule–fragment comparison corresponded to the highest Tanimoto similarity among the individual fragment–fragment comparisons. Here similarity was measured using Molecular Access System (MACCS) fingerprints, and was kept in cell W ij . MACCS keys are a set of questions about a two-dimensional structure, and are thus useful to capture chemical features beyond simple topological matching. Using MACCS fingerprinting, we increased the power to detect relevant features, while diminishing the sparseness of W . Then, the width of W was shrunk using statistical filtering. In the resulting matrix W LC , for each column j , rows displaying a MACCS similarity >0.8 were counted, and the significance of the over-representation of fragment j among molecules related to the disease was assessed using a right-tailed Fisher’s exact test. Please note that the contingency table classifies ‘positives’ and ‘unknowns’ (instead of ‘negatives’): this reduces statistical power, but should not affect the true positive rate ( Supplementary Fig. 11 ). Those fragments with a P -value<0.1 were retained [25] . Note that the selection of LC fragments underwent a final step that ensured an acceptable tradeoff between classification performance and statistical signal (see Data balancing below). From LC fragments, we selected a subset of HC representatives. In W , these had to elicit an odds ratio ≥10, a minimum support of three molecules and a Benjamini–Hochberg adjusted P -value <0.01. To report a diverse and representative set, we grouped those fragments that occurred in the same molecules. From each group, the fragment associated with more diseases was kept. Data balancing In general, few chemicals are known per disease, whereas the majority of chemicals is not related to it. We balanced W LC using a combination of under-sampling and SMOTE over-sampling [61] , [62] . For each case in the minority class (that is, chemicals annotated with a disease of interest), five new examples were created, up to a maximum of 1,000 instances. The majority class (that is, ‘unknown’ cases) was under-sampled to achieve a 1:1 proportion with the minority class. Then, columns in the balanced data set ( W LC′ ) were hierarchically clustered using Fastcluster [63] , and branches were pruned using DynamicTreeCut [64] with a minimum cluster size of 1. Inside each cluster, fragments were compared all-against-all to detect parent–child relationships. For a lineage of fragments, the one with the best initial over-representation P -value was retained. Overall, this led to matrices W LC′′ that had an even sampling through the rows and a simplified set of LC over-represented fragments in the columns. Chemical classifiers W LC′′ matrices above are suitable for machine learning because they have a balanced class distribution, and a representative and reasonably distinct set of variables. Given its general robustness in the learning of structure–activity relationships [65] , we chose to build chemical classifiers with the RF algorithm. For this, we used the randomForest R-package [66] , growing 10,000 trees and taking default values for the rest of parameters. As each tree returns a decision, class probabilities were estimated from voting. As schemed in Fig. 6 , we performed a stratified tenfold cross-validation of predictive models. Test and training sets were split before the LC fragment mining step (that is, before the variable selection, and therefore previous to the data balancing). Performance metrics in Table 1 were obtained from the reassembled vector of test predictions. Disease network construction In a chemo-centric disease network, disease A is linked to disease B if molecules annotated to A are predicted to relate with B . As we obtained M and T models, we can propose, at least, three different networks ( Fig. 5a and Table 2 ): (i) a comorbidity network, that links A to B if chemicals that cause A are predicted to cause B ; (ii) a drug repositioning network, where chemicals employed to treat A may also be useful to treat B and (iii) a drug side effect network that relates A to B when chemicals used in the treatment of A could cause B . To infer an edge from A to B , we tested A curated chemicals together with a set of chemicals unrelated to A and B using the B RF classifier. The strength of the association was assessed with the AUC of the cross-classification ROC plot, where molecules predicted to associate with B are checked for their association with A . Note that we removed easy cases by discarding disease pairs in the same branch of the medical hierarchy. To mine the examples discussed in Fig. 5 , we only considered those pairs that shared no chemicals, highlighting the importance of the fragment mining procedure. Network analysis Comparison of the comorbidity network with a clinical disease co-occurrence network: a clinical disease network was obtained from Hudine [38] , a comorbidity network that reports the RR of experiencing a disease when another disease is diagnosed. In Hudine, clinical reports are stored using the International Classification of Diseases, 9th revision (ICD-9). The mapping between MeSH and ICD-9 (three-digit code) terms was achieved using BioPortal’s (http://bioportal.bioontology.org) Unified Medical Language System (UMLS) concepts, and by best-matching MeSH and ICD-9 UMLS concepts with the UMLS-similarity Perl-package [67] (vector relatedness>0.8). We assigned a significance P -value to the coincidence between our chemo-centric network and Hudine comorbidities (RR≥20 or φ ≥0.06) [38] by using a right-tailed Fisher’s exact test. The corresponding confusion matrix classified predicted and unpredicted pairs, and pairs that were mapped and not mapped to Hudine. To demonstrate the need for robust disease models, we also built a comorbidity network (same ( A ) and ( B ) sets) that linked A to B simply if at least 50% of A LC fragments were LC fragments of B . In addition to a reduction in the number of edges of two orders of magnitude, we observed no significant coincidence with the clinical network. Comparison of the drug repositioning network with a drug repositioning network derived from known drugs: disease–disease associations were inferred based on drug indications [42] . For a pair of diseases A and B , we filled a 2 × 2 confusion matrix counting the number of drugs that are used to treat both, one or none of the diseases [68] . From this matrix, we obtained the two-tailed P -value of a Fisher’s test and the Matthews correlation coefficient. A and B were linked in the drug repositioning network if P -value ≤0.05 and Matthews correlation coefficient ≥0.15 (ref. 68 ). Like above, node mapping was achieved using UMLS term similarities, and the significance of the overlap with our results was evaluated analogously. Here again, we checked that the modelling step was important to provide significant results. Comparison of the side effect network with side effects reported in drug labels: we collected a side effect network from ref. 68 . This network represents side effects that occur frequently among approved drugs prescribed for a particular disease. As done for the comorbidity and the drug repositioning networks, we analysed its coincidence with our chemo-centric map, and confirmed the convenience of disease models for building the network. How to cite this article: Duran-Frigola, M. et al. A chemo-centric view of human health and disease. Nat. Commun. 5:5676 doi: 10.1038/ncomms6676 (2014).